Transcriptional activation by the thyroid hormone receptor through ligand-dependent receptor recruitment and chromatin remodelling A bimodal switch model is widely used to describe transcriptional regulation by the thyroid hormone receptor (TR). In this model, the unliganded TR forms stable, chromatin-bound complexes with transcriptional co-repressors to repress transcription. Binding of hormone dissociates co-repressors and facilitates recruitment of co-activators to activate transcription. Here we show that in addition to hormone-independent TR occupancy, ChIP-seq against endogenous TR in mouse liver tissue demonstrates considerable hormone-induced TR recruitment to chromatin associated with chromatin remodelling and activated gene transcription. Genome-wide footprinting analysis using DNase-seq provides little evidence for TR footprints both in the absence and presence of hormone, suggesting that unliganded TR engagement with repressive complexes on chromatin is, similar to activating receptor complexes, a highly dynamic process. This dynamic and ligand-dependent interaction with chromatin is likely shared by all steroid hormone receptors regardless of their capacity to repress transcription in the absence of ligand. Synthetic thyroid hormones are one of the most prescribed drugs worldwide to treat hypothyroidism. The thyroid hormone receptor (TR) belongs to the steroid hormone receptor family and exists as two different subtypes (TRα and TRβ) encoded by different genes and each in multiple thyroid hormone (T3)-binding and non-T3-binding isoforms [1] . Each subtype is expressed in a tissue-specific manner. TRβ1 is predominantly expressed in kidneys, liver, brain, heart and thyroid, while TRα is expressed at highest level in brain [1] . For simplicity, we will refer to T3-binding TR isoforms in the liver as TR. TR shares many structural and functional similarities with other members of the receptor family. However, in contrast to receptors such progesterone receptor (PR) and glucocorticoid receptor (GR), unliganded TR localizes primarily to the nucleus [2] and interacts with nucleosome-embedded DNA [3] . Unliganded, chromatin-bound TR represses transcription through direct interaction with transcriptional co-repressors such as SMRT and NCoR [4] , [5] , [6] . Binding of hormone is thought to induce a conformational change of TR, causing displacement of co-repressors and recruitment of co-activators [7] , [8] , [9] , [10] . This relatively simple bimodal switch, initially described in the late nineties, results in a transition from gene repression to gene activation [11] . Currently, this model is generally accepted for a basic understanding of TR-regulated gene transcription (for recent reviews see, for example, refs 12 , 13 , 14 ) and also discussed as a general principle for nuclear receptors and other transcription factors (TFs) [15] , [16] . We have previously shown that genomic scale studies using a combination of DNase-seq and chromatin immunoprecipitation sequencing (ChIP-Seq) inform our understanding of steroid hormone receptors interaction with chromatin [17] , [18] , [19] , [20] ; however, such data is currently unavailable for endogenous TR. Here we use ChIP-seq to identify endogenous TR-binding sites (TRBS) genome wide in mouse liver tissue and DNase-seq to map chromatin remodelling promoted by thyroid hormone. We confirm that the unliganded TR indeed interacts with a number of regions in the genome. However, in contrast to the bimodal switch model, we find evidence for considerable ligand-dependent TR recruitment to the genome and de novo remodelling of chromatin. Importantly, many thyroid hormone-regulated genes are associated with this mechanism of action. Moreover, in disagreement with models depicting TR as a repressor constitutively bound to chromatin in the absence of hormone, we find little evidence for TR footprints (FPs) genome wide, either in the presence or absence of ligand, suggesting that TR interaction with chromatin is generally highly dynamic. Thus, in addition to the ligand-dependent switch of transcriptional co-regulators recruited to chromatin-bound TR, we propose a model wherein TR is able to dynamically bind and increase accessibility of chromatin in a ligand-dependent manner. Thyroid hormone regulation of chromatin accessibility To understand the molecular consequences of genome-wide interaction of TR with chromatin, we mapped the DNase I accessible chromatin landscape in liver from mice treated with propylthiouracil (PTU) mimicking hypothyroid conditions and PTU followed by L-triiodothyronine (T3) resembling hyperthyroidism. Nuclei were purified from freshly isolated livers and treated with DNase I as previously described [21] . 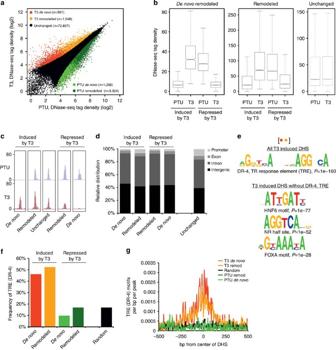Figure 1: Thyroid hormone inducesde novoremodelling of chromatin in the liver. (a) DNase-seq tag density of accessible chromatin in liver of mice treated with PTU or PTU together with T3. Replicate concordant DHS hotpots were identified based on two biological replicates (average tag densities of DHSs from the two biological replicates are plotted). Red and orange data points represent DHS hotspots increased in accessibility as a consequence of T3 treatment, where red marksde novoDHSs. Dark and light green represent DHS hotspots with decreased accessibility after T3 treatment, where light green marks DHS that disappears as a consequence of hormone treatment. Black shows unchanged accessible regions. Differential DHS accessibility where identified at an adjustedPvalue<0.05. (b) Distribution of DNase-seq tag density atde novo, remodelled and unchanged accessible regions. (c) Representative genome browser shots of DHS categorized asde novo, remodelled and unchanged. (d) Relative distribution of DHS within promoters (−1 kb to +100 bp of TSS), exons, introns and intergenic regions. (e) Upper panel,de novomotif analysis of all DHS with T3-induced DNase accessibility. The most enriched motif is shown. Lower panel,de novomotif analysis of T3-induced DHS lacking the identified canonical DR4-based thyroid hormone response elements (TRE). The three most enriched motifs are shown. (f) Frequency of the DR4 TRE at T3-induced and repressed accessible regions of chromatin. (g) Relative distribution of DR4 TRE in DHS hotspots, where accessibility is T3 regulated. Small mildly digested DNA fragments liberated from accessible chromatin were purified by sucrose gradients and initially sequenced to a depth of 20–30 million tags ( Supplementary Table 1 ). Replicate concordant DNase hypersensitive sites (DHS) were identified as previously described [17] ; between 65,000 and 73,000 DHSs were mapped in liver from hypo and hyperthyroid animals. Interestingly, we find thousands of regions where T3 treatment results in robust changes of chromatin accessibility ( Fig. 1a ). Sixty-nine per cent of the changes are modest but significant (remodelled DHS, Fig. 1a,b ) and likely reflect a net gain or loss of TFs or a transition of co-regulator interaction with TFs at the individual remodelled regions. Importantly, in contrast to the current model of constitutive TR interaction with chromatin, we observe that 31% of the differentially regulated DHSs are either formed or erased, where half of these are generated de novo as a consequence of T3 treatment ( de novo , Fig. 1a,b ). Figure 1c illustrates representative categories of accessible regions of chromatin identified. The hormone-remodelled regions are primarily located within intronic and intergenic regions ( Fig. 1d ) in agreement with genome-wide hormone-dependent chromatin remodelling by other steroid hormone receptors [18] . De novo motif analysis of DHSs induced by T3 shows an enrichment of a DR4-like motif ( Fig. 1e ) closely resembling the canonical DR4-based TR response element (TRE) and matches the TRE reported recently based on ChIP-seq against tagged overexpressed TR [22] , [23] , [24] . In addition to the TRE, we also find enrichment of motifs for HNF6 and FOXA. We do not find any additional significant enrichment of palindromic or inverted repeats of the AGGTCA half site. Approximately half of the remodelled DHSs contain the DR4-based TRE ( Fig. 1f ), suggesting that TR directly interacts with DNA at these sites. Thus at de novo- remodelled TREs, TR may be ligand dependently recruited to chromatin. In contrast, the DHSs with T3-dependent reduced accessibility are not enriched for DR4 TRE motifs compared with unchanged accessible regions ( Fig. 1f,g ), implying either that TR is not interacting directly with DNA at these sites and they are remodelled by secondary factors or that TR is recruited by a mechanism independent of the DR4 motif. At the T3-reduced DHS, we found enrichment of motifs likely to bind a number of liver-enriched transcriptions factors such as HNF4, C/EBP and HNF1 ( Supplementary Fig. 1a ). Figure 1: Thyroid hormone induces de novo remodelling of chromatin in the liver. ( a ) DNase-seq tag density of accessible chromatin in liver of mice treated with PTU or PTU together with T3. Replicate concordant DHS hotpots were identified based on two biological replicates (average tag densities of DHSs from the two biological replicates are plotted). Red and orange data points represent DHS hotspots increased in accessibility as a consequence of T3 treatment, where red marks de novo DHSs. Dark and light green represent DHS hotspots with decreased accessibility after T3 treatment, where light green marks DHS that disappears as a consequence of hormone treatment. Black shows unchanged accessible regions. Differential DHS accessibility where identified at an adjusted P value<0.05. ( b ) Distribution of DNase-seq tag density at de nov o, remodelled and unchanged accessible regions. ( c ) Representative genome browser shots of DHS categorized as de novo , remodelled and unchanged. ( d ) Relative distribution of DHS within promoters (−1 kb to +100 bp of TSS), exons, introns and intergenic regions. ( e ) Upper panel, de novo motif analysis of all DHS with T3-induced DNase accessibility. The most enriched motif is shown. Lower panel, de novo motif analysis of T3-induced DHS lacking the identified canonical DR4-based thyroid hormone response elements (TRE). The three most enriched motifs are shown. ( f ) Frequency of the DR4 TRE at T3-induced and repressed accessible regions of chromatin. ( g ) Relative distribution of DR4 TRE in DHS hotspots, where accessibility is T3 regulated. Full size image T3 regulates transcription and local chromatin remodelling The findings shown in Fig. 1 clearly reveal that we have identified a number of regulatory regions in the genome that are dramatically remodelled by T3 treatment. To investigate whether these remodelled regions are relevant for T3-regulated gene transcription, we identified T3-regulated genes in liver under hypo or hyperthyroid conditions. Genome-wide regulation of T3-dependent transcription was analysed by Illumina expression arrays. We identified several known direct targets of TR such as Thrsp/Spot14 and Dio1 (arrows, Fig. 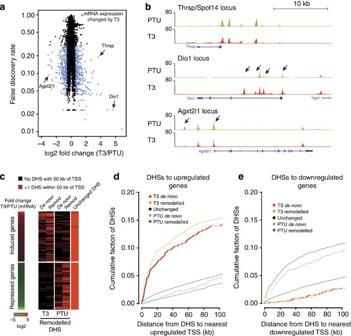Figure 2: Chromatin remodelling correlates with level of nearby gene transcription. (a) T3-induced and -repressed genes in the liver identified by mRNA expression microarrays of three independent biological repeats. Blue data points represent differentially expressed genes scored by an FDR of 0.3 and a log2 fold change of 1.5 (genes induced by T3) or −1.5 (genes repressed by T3). Two T3-induced genes (ThrspandDio1) and one T3-repressed gene(Agxt2l1) are marked by arrows. (b) Level of DNase accessibility near regions of T3-induced genes (ThrspandDio1) and a repressed gene(Agxt2l1). Arrows mark DHS accessibility regulated by T3. (c) Heatmap illustrating quantity of T3-regulated genes with at least one T3-regulated DHS within 50 kb of TSS. Genes are sorted from most induced to most repressed by T3. (d) Cumulative fraction of T3-regulated DHS near TSS (0–100 kb) of T3-induced genes. (e) Cumulative fraction of T3-regulated DHS near TSS (0–100 kb) of T3-repressed genes. 2a and Supplementary Table 2 ). We found no apparent changes of chromatin accessibility of regulatory regions near Thrsp ( Fig. 2b , upper panel), a well-described target for TR in liver, consistent with co-factor switching as the mechanism of TR activity at this locus. Interestingly, however; transcriptional induction of Dio1 is associated with de novo and induced remodelling of several regulatory sites near the Dio1 promoter ( Fig. 2b , middle panel). In fact, a significant number of T3-induced genes were associated with nearby T3-remodelled chromatin compared with T3-repressed genes ( Fig. 2c ) and more than half of T3-induced genes but less than a tenth of T3-repressed genes have at least one induced remodelled DHS region within 50 kb of the transcription start site (TSS) ( Supplementary Fig. 1b ). Also regions with increased accessibility after T3 treatment were significantly closer to TSSs of T3-induced genes compared with repressed DHSs ( Fig. 2d,e ). In contrast, T3-repressed genes, such as Agxt2l1 , are more frequently associated with DHSs reduced in accessibility after T3 treatment ( Fig. 2b,c and e and Supplementary Fig. 1b–d ). Thus, TR regulation of gene expression was to a large extent associated with nearby remodelling, including de novo remodelling, of regulatory regions, suggesting that the transition from repressed to activated state might not simply work through a switch from co-repressor to co-activator interaction with pre-occupied TR. In addition, co-activators and chromatin remodellers may also be recruited through ligand-dependent TR occupancy of chromatin, a mechanism shared with other steroid hormone receptors such as GR, PR and AR. Figure 2: Chromatin remodelling correlates with level of nearby gene transcription. ( a ) T3-induced and -repressed genes in the liver identified by mRNA expression microarrays of three independent biological repeats. Blue data points represent differentially expressed genes scored by an FDR of 0.3 and a log2 fold change of 1.5 (genes induced by T3) or −1.5 (genes repressed by T3). Two T3-induced genes ( Thrsp and Dio1 ) and one T3-repressed gene (Agxt2l1 ) are marked by arrows. ( b ) Level of DNase accessibility near regions of T3-induced genes ( Thrsp and Dio1 ) and a repressed gene (Agxt2l1 ). Arrows mark DHS accessibility regulated by T3. ( c ) Heatmap illustrating quantity of T3-regulated genes with at least one T3-regulated DHS within 50 kb of TSS. Genes are sorted from most induced to most repressed by T3. ( d ) Cumulative fraction of T3-regulated DHS near TSS (0–100 kb) of T3-induced genes. ( e ) Cumulative fraction of T3-regulated DHS near TSS (0–100 kb) of T3-repressed genes. Full size image Identification of TRBS in liver tissue To evaluate actual TR recruitment to chromatin genome wide at regions remodelled by T3, we applied ChIP-seq against endogenous TR. We used an in-house produced monoclonal antibody against the ligand-binding domain of TRβ (TR antibody C1). This antibody recognizes both TRβ and TRα ( Supplementary Fig. 2 ). However, only TRβ, but not TRα1 was detected in liver nuclear extracts by co-IP experiments ( Supplementary Fig. 2a ). To reduce the number of false positives in our ChIP-seq for TRBS, we performed a parallel ChIP-seq against TR in livers from mice with deficiency in both TR isoforms (TR double knockout (KO) mice). Enriched regions for TR occupancy were subsequently identified using TR double KO as background control and a stringent cutoff criterion for peak identification. We identified 864 TRBS under hypothyroid conditions and 2,186 under hyperthyroid conditions ( Fig. 3a ). Most ligand-independent TR peaks overlapped with TR peaks identified in presence of T3, generating a group of 651 preexisting TRBS. More than twice as many ligand-facilitated TRBS were found. De novo motif analysis of TRBS shows enrichment of the TRE closely resembling the TRE identified within T3-remodelled DHS (compare top panels of Figs 3b and 1e ). Close to 60% of the preexisting and 42% of the hormone-facilitated TRBSs contain TREs (bottom panel, Fig. 3b ), whereas <20% of the TRBSs unique to hypothyroid conditions contain a TRE, which is close to background levels of TREs in accessible chromatin (broken line in the bottom panel of Fig. 3b ). The tag density of the TRBSs unique to hypothyroid conditions is also significantly lower than preexisting TRBSs ( Supplementary Fig. 3a ), suggesting that these peaks may either be indirect TRBSs (that is, tethered to other TFs) or false positives. In general, 92% of TRBSs localize to accessible chromatin ( Supplementary Fig. 3b ), in agreement with previous reports on steroid hormone receptor occupancy of the accessible genome [17] , [18] , [25] . 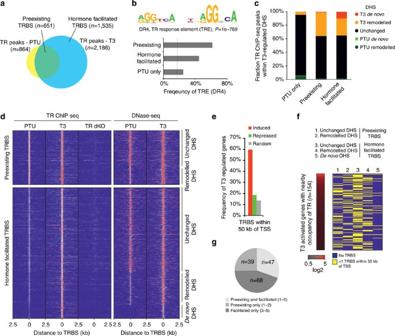Figure 3: Thyroid hormone-induced chromatin remodelling correlates with hormone-induced TR occupancy. ChIPs were performed on livers from mice treated with PTU, PTU+T3 and TR dKO. TR-binding sites (TRBS) were identified using HOMER with the TR ChIP-seq in TR dKO as a background control, a FDR threshold of 0.001 and a tag density threshold of 10 tags per peak. (a) The Venn diagram illustrates the overlap of TRBS in livers of PTU (yellow) and PTU plus T3-treated (blue) mice. Preexisting TR binding was defined by presence of TR peaks in absence and presence of T3, whereas hormone-facilitated TR binding was defined by a TR peak unique to T3 treatment. (b) Top panel,de novomotif analysis of TRBS in presence of T3. The most enriched motif is shown. Bottom panel, frequency of identified TRE in preexisting, hormone-facilitated and hormone-depleted TRBS. Broken line represents frequency of the TRE in all DNase-accessible regions of the genome in liver. (c) Distribution of TRBS within DHS regulated by T3 treatment. (d) Heat map illustrating TR ChIP-seq and DNase-seq tag distribution surrounding TRBS within the different categories of unchanged and T3-induced DHS. (e) Frequency of T3-regulated genes with at least one TRBS within 50 kb of TSS. Two hundred TSS from random genes were chosen as background control. (f) Heat map illustrating quantity of T3-activated genes with at least one TRBS (category 1–5) within 50 kb of TSS. Following TRBS categories are quantified: (1) Preexisting TRBS within unchanged DHS. (2) Preexisting TRBS within remodelled TRBS. (3) Hormone-facilitated TRBS within unchanged DHS. (4) Hormone-facilitated DHS within remodelled DHS. (5) Hormone-facilitated TRBS withde novoremodelled DHS. Genes are sorted from most induced and to most repressed by T3. (g) Number of T3-activated genes with a preexisting TRBS (n=39, 25%), hormone-facilitated TRBS (n=68, 44%) or a combination of preexisting and hormone-facilitated TRBS (n=47, 31%) within 50 kb of TSS. Figure 3: Thyroid hormone-induced chromatin remodelling correlates with hormone-induced TR occupancy. ChIPs were performed on livers from mice treated with PTU, PTU+T3 and TR dKO. TR-binding sites (TRBS) were identified using HOMER with the TR ChIP-seq in TR dKO as a background control, a FDR threshold of 0.001 and a tag density threshold of 10 tags per peak. ( a ) The Venn diagram illustrates the overlap of TRBS in livers of PTU (yellow) and PTU plus T3-treated (blue) mice. Preexisting TR binding was defined by presence of TR peaks in absence and presence of T3, whereas hormone-facilitated TR binding was defined by a TR peak unique to T3 treatment. ( b ) Top panel, de novo motif analysis of TRBS in presence of T3. The most enriched motif is shown. Bottom panel, frequency of identified TRE in preexisting, hormone-facilitated and hormone-depleted TRBS. Broken line represents frequency of the TRE in all DNase-accessible regions of the genome in liver. ( c ) Distribution of TRBS within DHS regulated by T3 treatment. ( d ) Heat map illustrating TR ChIP-seq and DNase-seq tag distribution surrounding TRBS within the different categories of unchanged and T3-induced DHS. ( e ) Frequency of T3-regulated genes with at least one TRBS within 50 kb of TSS. Two hundred TSS from random genes were chosen as background control. ( f ) Heat map illustrating quantity of T3-activated genes with at least one TRBS (category 1–5) within 50 kb of TSS. Following TRBS categories are quantified: (1) Preexisting TRBS within unchanged DHS. (2) Preexisting TRBS within remodelled TRBS. (3) Hormone-facilitated TRBS within unchanged DHS. (4) Hormone-facilitated DHS within remodelled DHS. (5) Hormone-facilitated TRBS with de novo remodelled DHS. Genes are sorted from most induced and to most repressed by T3. ( g ) Number of T3-activated genes with a preexisting TRBS ( n =39, 25%), hormone-facilitated TRBS ( n =68, 44%) or a combination of preexisting and hormone-facilitated TRBS ( n =47, 31%) within 50 kb of TSS. Full size image Although we used stringent criteria for TR peak identification the number of identified TRBS is relative low compared with other nuclear receptors in mouse liver tissue (for example GR>10,000 binding sites [17] ). Moreover, the detected TR only occupy 27% of the total T3 remodelled and 14% of the de novo -remodelled DHS ( Supplementary Fig. 3c ), collectively implying that the monoclonal TR antibody used here could fail to immunoprecipitate the total pool of TR bound to chromatin. To confirm TR occupancy of chromatin, we probed genome-wide binding of RXRα, reported to be the most frequent heterodimerization partner of TR in liver [26] . A total of 41% of T3-remodelled DHS and 24% of T3 de novo -remodelled chromatin is occupied by RXR ( Supplementary Fig. 3c ), suggesting that the monoclonal TR antibody may miss a subpopulation of potential TRBS. However, the overall RXR ChIP-seq tag density of the RXR-binding sites not occupied by TR is significantly lower compared with TR-RXR co-occupied sites ( Supplementary Fig. 3d ), suggesting that the TR antibody fails to detect these potential binding sites as a result of low receptor occupancy and less likely due to possible epitope masking. Moreover, the TRE frequency is considerably lower at T3-remodelled DHS occupied by RXR without TR compared with RXR sites co-occupied by TR ( Supplementary Fig. 3e ), suggesting that many of the potential additional TRBS identified using RXR ChIP-seq may be weak indirect TRBS from tethering to other TFs. Thus chromatin in liver tissue may indeed harbour a relative low number of TRBS. In agreement, <5,000 TR molecules per cell has been estimated to be expressed in murine liver tissue [27] in contrast to, for example, >60,000 GR molecules per cell in liver [28] , suggesting that the relative low number of TRBS reflects low abundance of the receptor. In addition, recent studies probing dexamethasone-dependent GR occupancy of accessible chromatin in liver tissue using a combination of three different antibodies also demonstrates a relative low frequency of de novo -remodelled DHS occupied by GR (13%) at a given point of time [17] . Importantly, similar trends are seen for ER and AR occupancy of remodelled chromatin in MCF7 and LNCaP cells, respectively [25] , inferring that low receptor occupancy of remodelled DHS is not necessarily a technical issue related to the antibody but may be associated to the dynamic behaviour of nuclear receptors (see below) or secondary effects of hormone treatment. T3-dependent and independent TR occupancy of chromatin The presented DNAse-seq and ChIP-seq against endogenous TR implies considerable ligand-dependent recruitment of TR to chromatin. Preexisting and hormone-facilitated TRBS are primarily located within unchanged and differentially remodelled DHS and almost no TR binding is found within DHSs reduced in accessibility as a consequence of T3 treatment ( Fig. 3c ). Interestingly, 10% of hormone-facilitated TR recruitment localize to de novo -remodelled chromatin, demonstrating that ligand-dependent TR recruitment to chromatin may function to regulate access to the chromatinized DNA template at a subset of TRBS ( Fig. 3c ). Since the vast majority of TRBS are found within unchanged and T3-induced accessible DHSs, we divided TRBS into hormone-preexisting and -facilitated binding sites and subdivided each group according to interaction with unchanged or induced DHSs ( Fig. 3d ). 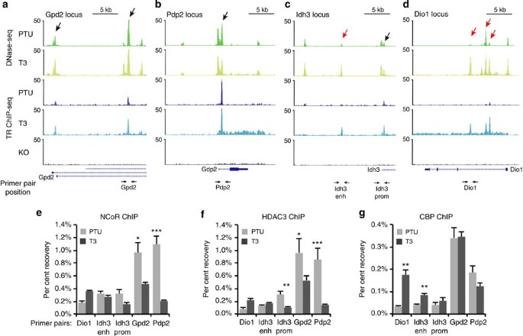Figure 4: Recruiment of co-repressors and co-activators to ligand-dependent and ligand-independent TRBS. (a–d) Examples of T3-activated genes (Idh3,Gpd2,Dio1andPdp2) harbouring nearby TRBS with preexisting TR occupancy (black arrows) and hormone-facilitated TR occupancy (red arrows). (e–g) ChIP against NCoR (e), HDAC3 (f) and CBP (g) at TRBS indicated ina–d. ChIPs were performed on livers from mice treated with PTU and PTU+T3. Error bars indicate s.e.m. withn=4 in each group. *P<0.05. **P<0.01. ***P<0.001 (t-test). Supplementary Figure 4a shows overall DNase-seq tag density of the different types of TRBS. Very few de novo DHSs was identified within preexisting TRBS, illustrating that unliganded TR primarily occupies accessible chromatin. Interestingly, within all groups of TRBS, T3 increases overall TR recruitment to chromatin, even though it is most pronounced at the hormone-facilitated TRBS ( Supplementary Fig. 4b ). Also the TR ChIP-seq signal in hypothyroid condition is higher within preexisting TRBS compared with hormone-facilitated TRBS ( Supplementary Fig. 4b ). Similar observation is seen for RXR ChIP-seq signal at TRBS occupied by RXR ( Supplementary Fig. 4c ). This demonstrates that hormone generally stimulates TR occupancy of chromatin, which agrees with recent reports showing hormone-facilitated recruitment of ectopically expressed TR [22] . Interestingly, T3 does not lead to increased TR accumulation in the nucleus ( Supplementary Fig. 2a ), suggesting that increased chromatin occupancy is not simply explained by increased protein concentration. To identify potential mechanisms regulating selective TR recruitment to preexisting TRBSs and insignificant binding to hormone-facilitated TRBSs in hypothyroid condition, we mined the TRBSs for enrichment and motif strength of the DR4 element identified. Interestingly, TRBSs within accessible chromatin bound by unliganded TR have a higher frequency of TRE and higher TRE motif score ( Supplementary Fig. 5a,b , orange) compared with accessible TRBS not bound by unliganded TR ( Supplementary Fig. 5a,b , grey). Also, TRBSs bound by unliganded TR have a higher degree of accessibility in hypothyroid condition compared with unbound accessible TRBSs ( Supplementary Fig. 5c ). Notably, de novo remodelled TRBSs have the highest frequency of TREs and the highest TRE motif score ( Supplementary Fig. 5a,b , red). Thus, selective TR recruitment to chromatin is determined by the strength and frequency of the response element. Here unliganded TR preferentially occupies accessible chromatin with a strong consensus motif. Less accessible chromatin with weaker binding motifs display low occupancy by TR. Interestingly, a highly conserved motif is needed at sites where TR is able to penetrate inaccessible chromatin. Binding leads to remodelling through recruitment of co-activator complexes. Consequently, unliganded TR will not occupy these types of response elements. T3-activated but not -repressed genes associated with TRBS To gain insight to the mechanism regulating TR-dependent gene transcription, we mapped TRBS in vicinity to T3-regulated genes. Sixty per cent of T3-induced genes have at least one TRBS within 50 kb of the TSS ( Fig. 3e ). In contrast, T3-repressed genes show little enrichment of nearby TRBS, suggesting that liganded TR is preferentially associated with gene activation ( Fig. 3e ). We observe a similar trend for a range of regions between 5 and 200 kb of TSS from T3-regulated genes ( Supplementary Fig. 5d ). This agrees with the absence of TR-binding motifs in T3-regulated DHS near T3-repressed genes ( Fig. 1e ). Collectively, 154 T3-activated genes have nearby occupancy of TR ( Supplementary Table 2 ). This list of genes likely constitutes direct TR targets in liver and gene ontology analysis indicates direct TR regulation of genes involved in fatty acid, steroid and cholesterol metabolism ( Supplementary Table 3 ). Interestingly, TR-activated genes have nearby binding of multiple different TRBS described above ( Fig. 3f ). Importantly, two-thirds of the T3-activated genes are associated with hormone-facilitated TR recruitment to chromatin ( Fig. 3g ), suggesting that hormone-facilitated recruitment of TR to chromatin contributes to the regulation of a majority of direct TR target genes. TR has been reported to bind DNA as a mono, homodimer or heterodimer with RXR [1] . RXRα co-occupies 72% of TRBS in hypothyroid condition and 60% of TRBS in hyperthyroid condition ( Supplementary Fig. 3f ), suggesting that the majority of TR interacts with chromatin as a heterodimer with RXRα. This observation contradicts recent TR ChIP-seq data using overexpression of TR, where <40% of TR was reported to overlap with RXR [22] . However, the study showed that TR co-occupancy of RXR had a higher correlation with nearby T3-regulated gene transcription compared with TRBS without RXR. In agreement, we also observed a higher frequency of T3-induced genes with nearby occupancy of TR-RXR compared with TRBS without presence of RXR ( Supplementary Fig. 5e ). Neither TR-RXR co-occupancy nor TR occupancy without RXR correlates with nearby repression, implying that TR homodimers are not specifically involved in gene repression. Activation of TR target genes through multiple mechanisms Idh3 , Gpd2 and Pdp2 represent direct TR target genes with nearby occupancy of TR in hypothyroid condition and thus potentially actively repressed by TR in that state ( Fig. 4a–c and Supplementary Table 2 ). In agreement, previous studies have shown that Idh3a is de-repressed in a TRβ KO model under hypothyroid condition [29] and mutation of NCoR-disrupting interaction with TR de-represses Gpd2 and Idh3a transcription in hypothyroid animals [30] . Activation of Gpd2 and Pdp2 transcription is not associated with considerable change of TR occupancy and chromatin is not significantly remodelled ( Fig. 4a,b ). At the Gpd2 and Pdp2 TRBSs, NCoR and HDAC3 occupancy is reduced in response to T3 ( Fig. 4e,f ); however, CBP is present at the TRBSs in the absence and the presence of ligand ( Fig. 4g ). This suggests that activation of Gpd2 and Pdp2 is coupled with co-repressor disassociation but in contrast to the bimodal switch model, co-activator pre-occupies TRBS in the absence of hormone and continues to occupy chromatin in the presence of hormone. Figure 4: Recruiment of co-repressors and co-activators to ligand-dependent and ligand-independent TRBS. ( a – d ) Examples of T3-activated genes ( Idh3 , Gpd2 , Dio1 and Pdp2 ) harbouring nearby TRBS with preexisting TR occupancy (black arrows) and hormone-facilitated TR occupancy (red arrows). ( e – g ) ChIP against NCoR ( e ), HDAC3 ( f ) and CBP ( g ) at TRBS indicated in a – d . ChIPs were performed on livers from mice treated with PTU and PTU+T3. Error bars indicate s.e.m. with n =4 in each group. * P <0.05. ** P <0.01. *** P <0.001 ( t -test). Full size image Idh3 represents a gene harbouring different types of TRBS in vicinity of the TSS ( Fig. 4c ). Close to the TSS, TR occupies a TRBS in the absence of hormone ( Fig. 4c , Idh3, promoter). In addition, at a 8 kb upstream TRBS TR is hormone dependently recruited to chromatin associated with increased chromatin remodelling ( Fig. 4c , Idh3 , enhancer). NCoR and HDAC3 dissociate from the promoter in response to T3 treatment ( Fig. 4e,f ) and CBP is recruited to the enhancer ( Fig. 4g ), illustrating that a combination of co-repressor loss at one site and co-activator gain at another site may drive activation of transcription. Interestingly, Dio1 represents a class of genes, where all nearby TR binding is ligand-dependent and TR recruitment leads to dramatic remodelling of the TRBSs ( Fig. 4d ). Presence of T3 leads to increased recruitment of co-activator CBP ( Fig. 4g ), whereas NCoR and HDAC3 occupancy remains unchanged at the TRBS ( Fig. 4e,f ). Thus, Dio1 is not a candidate for considerable direct repression by TR, concretely illustrating multiple mechanisms by which thyroid hormones regulate gene expression programmes. In agreement, disruption of NCoR–HDAC3 interaction have been reported to have little effect on Dio1 transcription in liver [31] . Absence of TR FPs within chromatin Early studies showed that at certain sites, liganded as well as unligand TR interaction with chromatin is associated with a DNase-accessible region and a FP corresponding to TR bound directly to DNA [3] . To gain genome-wide insight to direct TR interaction with chromatin within identified TRBS, we carried out deep sequencing (>100 million uniquely aligned tags) of DNase tag libraries from liver of hypo or hyperthyroid mice. Interestingly, we could not find evidence for significant genome-wide FPs protected from DNase cleavage at TR-bound TREs in comparison to unbound TREs ( Fig. 5a , top). Similarly, comparing the DNase cut profiles between the PTU and T3 conditions did not identify nuclease protection at preexisting TR-bound TREs ( Fig. 5b ). This indicates that the TR interaction with chromatin generally does not create a detectable TR FP. Moreover, the DNase cleavage pattern at the TRE is the same irrespective of TR presence or absence on chromatin and is essentially identical to the cleavage pattern for naked DNA ( Fig. 5a , bottom). This demonstrates that chromatin-bound TR does not leave a unique DNase cleavage signature and agrees well with recent findings, demonstrating that other steroid hormone receptors such as AR [32] , ER and GR [33] FP poorly and do not create DNase cleavage signatures different from DNase cleavage signatures on naked DNA. In contrast, and as a control for the DNase-seq quality, we found considerable protection from DNase cleavage at previously described ChIP-seq identified bindings sites for CTCF, E2F4 and several liver-enriched TFs, including C/EBP [34] ( Fig. 5c ). CTCF and C/EBP have previously been shown to FP genome wide [35] , [36] . Collectively, our findings demonstrate that TR occupancy is generally not associated with a FP in chromatin and this may likely be a general phenomenon for steroid hormone receptors irrespective of their ability to repress transcription. 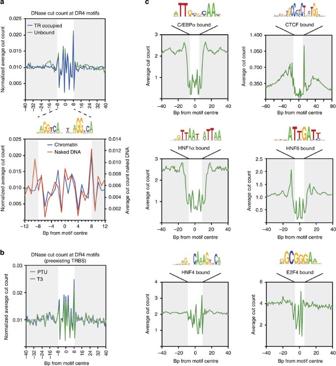Figure 5: Absence of DNase protection at DR4 motifs within TRBS. (a) Top panel, average DNase cut analysis of DR4 motifs enriched at TRBS within TR-bound (blue) and -unbound (green) regions of chromatin. DNase-seq library is from livers isolated from hyperthyroid mice. Average DNase cut count analysis of DR4 motifs at TR-bound (blue) and within genome-wide naked DNA from human IMR90 cells61(bottom panel). (b) Average DNase cut count analysis of DR4 motifs within preexisting pre-accessible TRBS under hypo (PTU, blue) or hyperthyroid (T3, green) condition. (c) Average DNase cut count analysis of motifs within C/EBPα, CTCF, HNF1A, HNF6, HNF4 and E2F4-binding sites identified previously in liver34. DNase-seq library is from livers isolated from hyperthyroid mice. Figure 5: Absence of DNase protection at DR4 motifs within TRBS. ( a ) Top panel, average DNase cut analysis of DR4 motifs enriched at TRBS within TR-bound (blue) and -unbound (green) regions of chromatin. DNase-seq library is from livers isolated from hyperthyroid mice. Average DNase cut count analysis of DR4 motifs at TR-bound (blue) and within genome-wide naked DNA from human IMR90 cells [61] (bottom panel). ( b ) Average DNase cut count analysis of DR4 motifs within preexisting pre-accessible TRBS under hypo (PTU, blue) or hyperthyroid (T3, green) condition. ( c ) Average DNase cut count analysis of motifs within C/EBPα, CTCF, HNF1A, HNF6, HNF4 and E2F4-binding sites identified previously in liver [34] . DNase-seq library is from livers isolated from hyperthyroid mice. Full size image Unlike steroid hormone receptors such as GR, AR and PR, unliganded TR is localized to the nucleus, where the receptor interacts with chromatin to repress transcription. Over the last two decades, transcriptional regulation by TR has been described by a model, wherein TR is bound to chromatin in the absence of ligand, recruits co-repressor complexes and represses transcription. On ligand binding, the receptor undergoes a hormone-dependent conformational change, leading to disassociation of co-repressors and recruitment of co-activators. This model originates from early pioneering studies on steroid hormone receptors, where TR was demonstrated to interact with chromatin both in the presence and the absence of hormone [37] , [38] . Interaction was shown to be associated with increased DNase hypersensitivity and bound TR was demonstrated to FP [3] , leading to the general assumption that TR is constitutively bound to chromatin. Subsequent identification of transcriptional co-activators and co-repressors interacting with TR led to the widely accepted co-factor switch model described above ( Supplementary Fig. 6a ). This predicts that genome-wide footprinting analysis may be used to identify TREs. Unexpectedly, we find that thyroid hormone induces a considerable number of genome-wide de novo DNase hypersensitive sites harbouring putative TRBS (DR4), indicating that TR can be recruited to chromatin in a ligand-dependent manner, resulting in a DNase hypersensitive site. ChIP-seq against endogenous TR supports a model where TR can be recruited to chromatin in a ligand-dependent manner ( Supplementary Fig. 6c,d ). Importantly, we show that induced chromatin remodelling, including de novo remodelling, is associated with thyroid hormone-induced (and not repressed) transcription of nearby genes, demonstrating that ligand-dependent recruitment of TR and resulting chromatin remodelling are associated with thyroid hormone-activated gene transcription. TR ChIP on a few promoters [39] and recent genome-wide ChIP-seq studies of exogenous expressed TR [22] , support our findings that TR can be recruited to chromatin in a ligand-dependent manner. Also, mutation of NCoR disrupting TR-NCoR interaction and mutation of NCoR abolishing HDAC3 interaction only leads to de-repression of a subset of TR-regulated genes [30] , [31] , and repression of positively regulated TR target genes is only observed for a subset of thyroid hormone-activated genes [29] . These findings collectively suggest an alternative mechanism for TR-regulated gene transcription, wherein ligand-dependent recruitment of TR to the genome can result in de novo remodelling of chromatin- and dynamic-assisted loading of transcriptional co-regulators [20] , [40] ( Supplementary Fig. 6d ). Notably, the previously described dynamic mobility of TR in living cells [41] is also supportive of the model described here. This mechanism is shared with a subset of GR, PR and AR chromatin interaction events [17] , [18] , [25] , [42] , [43] . Moreover, and in agreement with observations from other steroid hormone receptors [17] , repressed transcription as a consequence of hormone treatment is associated with nearby regions with reduced chromatin accessibility. These regions are not enriched for hormone receptor binding sites and are thus possibly regulated by indirect mechanisms such as transcriptional co-regulator sequestering. In addition, TR ChIP-seq does not show enrichment of TRBS near repressed genes in agreement with tagged TR ChIP-seq studies from neuronal cells [24] . A recent study using TR overexpression suggested that hormone-facilitated gene repression is linked to reduced TR occupancy [22] . We do not find significant reduction of endogenous TR occupancy in response to hormone. Although stable unliganded TR interaction with chromatin predominates in current models, several early studies indicated that TR does not necessarily FP on chromatin in the absence of ligand [44] , [45] . Using a genome-wide footprinting strategy, we show that, in contrast to several factors (for example, C/EBP and HNF6) TR generally does not footprint ( Fig. 5a,b ). Importantly, we did not find FPs at TRBS in the hypothyroid condition, suggesting that repressive TR interaction with chromatin is dynamic ( Supplementary Fig. 6b ). Lack of footprinting may be a general phenomenon for steroid hormone receptors [32] , [33] and may be credited to the highly dynamic mechanisms of their interaction with chromatin [20] , [33] , [41] , [46] . Collectively, we demonstrate that TR is recruited to chromatin by multiple mechanisms, including hormone-independent interactions with TREs for unliganded TR and ligand-induced TR recruitment to chromatin. This leaves a very important question of how TR discriminates between these two extremes, especially in hypothyroid conditions. Motif analysis suggests that the presence and strength of the TR-binding motif (DR4) within accessible chromatin is an important determinant regulating TR occupancy of chromatin in absence of T3, where unliganded TR preferentially occupy regions with strong TREs. In contrast, when T3 is available, TR is able to occupy accessible chromatin harbouring less stringent TR-binding motifs. Here ligand-facilitated recruitment to pre-accessible chromatin may be orchestrated by cooperation with pre-bound TFs [17] , [47] , [48] , [49] . Cooperation likely requires liganded TR and will only be favourable under such conditions. Alternatively binding to weak TREs may be regulated by nuclear distribution of TR. Previous studies have shown that hormone changes continuous shuttling of TR between cytoplasm and nucleus as well as redistribution of TR in the nucleus [2] , [41] . Reorganization of TR may increase subnuclear TR concentration and drive hormone-dependent recruitment to specific sites of the genome. Changing local TF concentration relative to the amount of binding sites have been shown to rewire transcriptional networks, likely determined by differential affinity of TF for its degenerated binding sequence [50] . Thus, binding of TR to particular TRBS may be driven by specific receptor–DNA affinity, and increasing TR concentration may therefore increase occupancy of particular hormone-sensitive TRBS. Such hormone-sensitive TRBS may work similar to the reported glucocorticoid hypersensitive sites [51] . Importantly, however, we do not observe considerable increase in nuclear accumulation of TRβ probed by IP ( Supplementary Fig. 2a ). Interestingly, at a subset of TRBS and in the presence of T3, TR is able to penetrate an inaccessible chromatin configuration and induce de novo chromatin remodelling. Here a strong TRE is required ( Supplementary Fig. 5b ) together with the ability to interact with transcriptional co-activators ( Fig. 4g ). Consequently, these TRBS cannot be accessed by unliganded TR. Selectivity to these sites may also be driven by cooperation with other TFs, and remodelling proteins to remodel chromatin and promote TR occupancy as seen for other steroid hormone receptors such as GR [17] , [25] , [49] , [52] . Collectively, this opens a series of new questions regarding specificity and importance of ligand-dependent TR binding to chromatin and may facilitate additional molecular insights into the basis of TR mutations in disease. Animal work Wild-type mice were treated with PTU (0.15%; Harlan Teklad, Cat#TD.95125) for 3 weeks and then divided into two groups. One group was treated with PTU to maintain hypothyroid status and the other group was treated with PTU together with i.p. injection of T3 injection at a dose of 10 μg per 100 g body weight for 5 days to make mice hyperthyroid. The animal study was carried out according to the protocol approved by the National Cancer Institute Animal Care and Use Committee. RNA expression analysis Total RNA (250 ng) was reverse transcribed priming with a T7 oligo(dT) primer, followed by second strand complementary DNA synthesis. Biotin-labelled complementary RNA was produced by in vitro transcription, and hybridized to MouseRef-8 v2.0 Expression BeadChip arrays according to the manufacturer’s instructions (Illumina). Three biological replicates (independent mice) were used for each condition (PTU and T3). RNA was hybridized to the Illumina MouseRef-8 v2.0 Expression BeadChip and raw data were extracted with Illumina BeadStudio software. Raw probe intensities were converted to expression values using the lumi package [53] in Bioconductor with background correction, variance stabilization by vst and quantile normalization. Differential expression between PTU and T3 conditions was assessed by an empirical Bayes analysis of a linear model using the limma package [54] in Bioconductor. False discovery rates were calculated with the Benjamini and Hochberg method, and differentially expressed genes were defined with a false discovery rate (FDR) cutoff of 0.3 and a fold change of 1.5. DNase digestion of chromatin Livers were isolated from mice and nuclei were immediately purified [21] and resuspended in buffer A (15 m M Tris-HCl pH 8.0, 15 m M NaCl, 60 m M KCl, 1 m M EDTA, 0.5 m M EGTA, 0.5 m M Spermidine and protease inhibitors) in a final concentration of 10 million nuclei per ml. DNase digestions were performed by adding 100 μl × 10 digestion buffer (60 m M CaCl 2 and 750 m M NaCl) containing various concentrations (0 U–100 U) of DNase I (Sigma). Digestions were incubated for 3 min at 37 °C and reactions were terminated by addition of one volume of stop buffer (50 m M Tris-HCl, 100 m M NaCl, 0.1% SDS, 100 m M EDTA and 50 μg ml −1 Proteinase K (Ambion)). Digested chromatin was incubated at 55 °C for 2 h and stored at 4 °C until further use. DNase I digestion efficiency was evaluated by quantitative PCR and samples with optimal digestion efficiency were incubated with 90 μg ml −1 RNase A (Sigma) for 30 min at 37 °C before 50–500 bp DNA fragments were purified using ultracentrifugation. Chromatin IP Frozen livers were homogenized in PBS containing 1% formaldehyde, incubated 10 min at room temperature and quenched with 0.125 M glycine. For HDAC3, CBP and NCoR IP’s an additional crosslinker, disuccinimidyl glutarate, was used prior to formaldehyde fixation. Crosslinked cells were washed in PBS, resuspended in lysis buffer (0.1% SDS, 1% Triton X-100, 150 m M NaCl and 20 m M HEPES pH 7.6) and sonicated using a Bioruptor (Diagenode). Chromatin was immunoprecipitated using monoclonal antibody C1 which preferentially recognize TRβ1, NCoR (Abcam, ab24552), HDAC3 (Santa Cruz, sc-11417), RXR (Santa Cruz, sc-553) and CBP (Santa Cruz, sc-369) and Protein A/G agarose beads (Santa Cruz, sc-2003) over night at 4 °C. IPs were performed in 1 ml aliquots using 3 μg of indicated antibodies. Immunocomplexes were washed extensively and chromatin was eluted and decrosslinked over night at 65 °C. DNA was subsequently phenol/chloroform purified and ethanol precipitated. Illumina sequencing ChIP- or DHS-isolated DNA (10 ng) was used in preparation of standard Illumina sequencing libraries. In brief, DNA fragments were end-repaired, adenylated and ligated to adapter sequences. Following gel purification, index sequences were introduced by PCR. Library cluster generation and single-end sequencing was performed on the Ilumina platform. Reads were aligned with bwa 0.5.9-r16 (ref. 55 ) to the mm9 reference genome and duplicates were marked with picard version 1.92 (ref. 56 ). DNase-seq and ChIP-seq analysis Replicate concordant DHS were identified using the Hotspot algorithm [57] . Differentially accessible DHS were scored using DESeq [58] from two biological replicates at adjusted P value<0.05. TR ChIP-seq enriched regions were identified by HOMER [59] using a TR ChIP-seq from TR KO as a background control, a FDR threshold of 0.1% and a tag density threshold of 10. RXR-ChIP-enriched regions were identified using input chromatin as control, a FDR threshold of 0.1% and a tag density threshold of 20. Enriched DNA motifs at DHS- and TR-enriched regions were identified using HOMER and heatmaps of ChIP-seq and DNase-seq data were generated using MeV [60] . Analysis of DNase protection at TF-binding sites From ultra deep sequencing of DNase-seq libraries, we generated DNase cut count profiles as described previously [35] . In short, because a single cut in a DNA segment by DNase I generates two end nucleotides, 5′ and 3′, we set the location to be the 5′ nucleotide to define cut count profile independently of the read strand from sequencing. If a read is mapped onto the forward strand, the cut site is defined as the −1 nucleotide (immediately 5′) from where the read starts. If a read is in the reverse strand, we define the cut site to be the first base of the read. Motifs within TF ChIP-seq peaks were extracted using HOMER and the average DNase cut count was evaluated at base pair resolution centred on TF motifs. Coordinates from liver-enriched TFs were based on previously published ChIP-seq data [34] . Accession codes : Gene expression microarray data have been deposited in the GEO database with accession number GSE65947 . ChIP- and DNase-sequencing data have been deposited in the SRA database with accession number SRP055020 . How to cite this article : Grøntved, L. et al. Transcriptional activation by the thyroid hormone receptor through ligand-dependent receptor recruitment and chromatin remodelling. Nat. Commun. 6:7048 doi: 10.1038/ncomms8048 (2015).